Adaptive real-time dual-comb spectroscopy The spectrum of a laser frequency comb consists of several hundred thousand equally spaced lines over a broad spectral bandwidth. Such frequency combs have revolutionized optical frequency metrology and they now hold much promise for significant advances in a growing number of applications including molecular spectroscopy. Despite an intriguing potential for the measurement of molecular spectra spanning tens of nanometres within tens of microseconds at Doppler-limited resolution, the development of dual-comb spectroscopy is hindered by the demanding stability requirements of the laser combs. Here we overcome this difficulty and experimentally demonstrate a concept of real-time dual-comb spectroscopy, which compensates for laser instabilities by electronic signal processing. It only uses free-running mode-locked lasers without any phase-lock electronics. We record spectra spanning the full bandwidth of near-infrared fibre lasers with Doppler-limited line profiles highly suitable for measurements of concentrations or line intensities. Our new technique of adaptive dual-comb spectroscopy offers a powerful transdisciplinary instrument for analytical sciences. Fourier transform spectroscopy [1] , [2] is the mature solution to a variety of problems [3] , [4] , [5] , [6] , [7] , [8] from the research laboratory to the manufacturing floor. The Michelson-based Fourier transform interferometer is known for more than 40 years as a benchtop instrument of great value in analytical sciences because it measures a broad range of optical frequencies simultaneously with accuracy and sensitivity. In recent years, novel techniques [9] , [10] , [11] , [12] , [13] , [14] , [15] , [16] , [17] , [18] , [19] , [20] , [21] , [22] , [23] , [24] , [25] , [26] , [27] , [28] , [29] , [30] , [31] have been developed in which a laser frequency comb [32] , [33] directly interrogates a vast number of transitions of a molecular sample. In particular, the precisely spaced spectral comb lines may be harnessed for dual-comb Fourier transform spectroscopy [14] , [15] , [16] , [17] , [18] , [19] , [20] , [21] , [22] , [23] , [24] , [25] , [26] , [27] , [28] , [29] , [30] , [31] . Dual-comb spectroscopy holds much promise for outperforming absorption measurements performed by Michelson-based Fourier transform spectroscopy: the recording time and resolution may be improved a million-fold, with potential broad spectral span in any spectral region. The technique may thus open up new opportunities for laboratory spectroscopy, as well as for field-based sensors. Furthermore, recent proof-of-principle experiments [29] , [30] , [31] demonstrate an intriguing potential for nonlinear multiplex spectroscopy, with possible applications ranging from microscopy [30] to sub-Doppler precision measurements [31] . However, the technique of dual-comb spectroscopy has not realized its full potential yet, mostly because of the difficulty of synchronizing the pulse trains of two comb lasers within interferometric precision. In this letter, we present a technique of real-time dual-comb spectroscopy that only requires free-running femtosecond oscillators and electronic signal processing, using commercially available components. Long measurement times, complex locking systems and computer algorithms are not needed. We demonstrate the suitability of our technique for the measurement of Doppler-broadened line profiles. We first explain the principle and challenges of dual-comb spectroscopy. We then describe a technique, which makes it possible to record real-time high-quality molecular spectra with free-running femtosecond lasers. We show its experimental performance with commercial fibre lasers emitting around 1.55 μm. We finally discuss its limitations as well as the new opportunities opened up by adaptive dual-comb spectroscopy. Stability requirements in dual-comb spectroscopy Dual-comb spectroscopy can be considered with the metaphor of a sampling oscilloscope. Pulses from comb 1 excite molecular free induction decay and pulses from comb 2 sample the waveform of this decay interferometrically. For simplicity, we at first ignore carrier–envelope phase shifts. At best, interferometric samples are taken at intervals 1/ f (for example, 10 −8 s) where f is the repetition frequency of comb 2 (for example, 100 MHz). If Δ f is the difference of comb repetition frequencies (for example, 100 Hz), consecutive interferometric samples result from pulse pairs showing a time separation increased by an amount Δ τ =Δ f / f 2 (for example, 10 −14 s). The ‘sampling oscilloscope’ thus effectively stretches the waveform of the free induction decay signal by a factor s = f /Δ f (for example, 10 6 ). Signal frequencies in this waveform are transformed down from the optical to the radio frequency region by the same factor s . In the experiment, the signal of the photodetector is electronically low-pass filtered to suppress the pulse repetition frequency f . The time-stretched waveform appears thus as a continuous electronic signal. This signal is digitized at a constant clock rate determined by the data acquisition board of the computer. For ideally stable frequency combs, the waveform thus sampled can be Fourier transformed to reveal the signal spectrum. In the real world, major difficulties arise from the residual instabilities of the frequency combs, even when these benefit from state-of-the-art stabilization. The time intervals between excitation and sampling pulses are indeed subject to some variations δ t , which appear in the detector signal stretched in time by the factor s . Let us now consider the slippage of the carrier phase relative to the pulse envelope owing to laser dispersion. If the carrier–envelope slippage frequencies of the two combs differ by f ce , the relative phases of pump and probe pulse will change by an additional 2π f ce / f between two interferometric samples, and all frequencies in the Fourier spectrum of the detector signal will be translated by f ce . As long as f ce is constant, the spectral translation can be accounted for if f ce is measured or if the absolute frequency of some spectral feature is known. Below, we describe an electronic signal processing technique that compensates for both timing fluctuations and phase fluctuations. In the frequency domain, dual-comb spectroscopy can be understood by considering the two frequency combs of slightly differing line spacing. The optical frequencies f n of a laser frequency comb may be written as f n = n f + f 0 , where n is a large integer and f 0 is the carrier–envelope offset frequency. Each pair of optical lines, one from each comb, produces a radio frequency beat note on the detector. These beat signals form a comb of radio frequencies f n ,rf = n Δ f + f ce . Optical frequencies are thus converted into radio frequencies with a conversion factor Δ f / f . The beat note between one pair of lines from the two combs must therefore be kept narrower than Δ f to preserve the resolution. Furthermore, for coherent measurement, the intrinsic linewidth of the beat note should be narrower than the inverse of the acquisition time. In other words, dual-comb spectroscopy requires interferometric short-term stability and the intrinsic noise of a radiofrequency-locked comb is significantly too high on times shorter than a millisecond [34] to allow for correct measurements. To record a distortion-free real-time interferogram, the jitters between subsequent pulses must be kept lower than 10 attoseconds. Otherwise, chromatic artefacts, called phase errors, spoil the spectrum [35] and cannot be accounted for a posteriori. These stability requirements are much more demanding than those for optical frequency metrology. There it is common practice to reference the comb to a stable microwave clock. Relatively slow servo loops of some kHz bandwidth are used to compensate for drifts of the pulse repetition frequency and the carrier–envelope offset frequency relative, and for shorter time scales, one relies on the intrinsic ‘flywheel’ stability of the laser [36] . Although the width of the comb lines remains typically on the order of 0.1–1 MHz under these circumstances, the effect of such short-term fluctuations becomes negligible for optical frequency measurements when averaging over times of seconds or minutes. Locking the comb to optical references makes it possible to achieve much narrower linewidths, but sub-Hz linewidth continuous-wave laser and fast feedback loop development require significant efforts that are not compatible with an easy-to-operate instrument. As a consequence, real-time dual-comb spectroscopy, allowing for distortion-free spectra of good quality Doppler-broadened line profiles and measurement times shorter than 1 s, remains challenging. Free-running or radiofrequency-locked combs yield artefacts and reduced signal-to-noise ratio [14] , [15] , [22] , [25] , [26] . Stabilizing the combs against state-of-the-art cavity-stabilized continuous-wave lasers with a hertz-level linewidth, far exceeding the stability available from common microwave oscillators, enables to record high-quality interferograms averaged over several seconds or minutes [16] , [19] , [20] , [23] . Such reports focused on long integration time (several minutes or more) for signal-to-noise ratio improvement and highly resolved comb lines. Possible phase errors in ms-timescale acquisitions might be thus cleaned up. Furthermore, this demanding approach can hardly be implemented outside the best frequency metrology laboratories. Alternatively, simultaneously recording the interferometric signal and the fluctuations of two loosely stabilized combs against two continuous-wave lasers to compute a posteriori corrections has been demonstrated [21] , [27] . This solution, with multiple data acquisition channels and computational treatment, also focused on its averaging capabilities, with continuous data acquisition and averaging during 24 h (Roy et al . [27] ). Principle of adaptive dual-comb spectroscopy In our technique of adaptive dual-comb spectroscopy ( Fig. 1 ), real-time compensation for the timing fluctuations and carrier–envelope phase shift variations is achieved by automatically triggering the data acquisition and correcting the interferometric signal with two adaptive signals. These signals are derived from two radiofrequency beat notes S 1 and S 2 , of frequency f a and f b , respectively, originating from different pairs of individual lines of the two different combs. 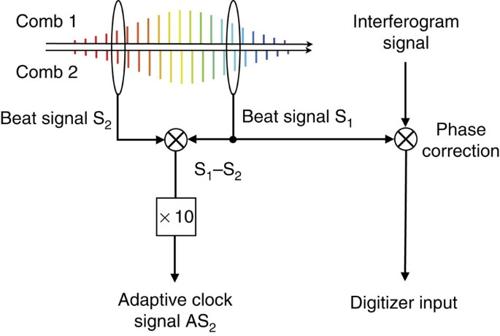Figure 1: Principle of adaptive dual-comb spectroscopy. Two radiofrequency beat notes S1and S2originating from different pairs of individual lines of the two different combs are generated simultaneously to the interferometric signal required for the spectroscopy experiment. The phase fluctuations of the interferometric signal are cancelled by electronic multiplication with the beat note signal S1. The difference between the beat signals S1and S2is only sensitive to timing variations and provides the clock signal AS2used for sampling the interferogram. Figure 1: Principle of adaptive dual-comb spectroscopy. Two radiofrequency beat notes S 1 and S 2 originating from different pairs of individual lines of the two different combs are generated simultaneously to the interferometric signal required for the spectroscopy experiment. The phase fluctuations of the interferometric signal are cancelled by electronic multiplication with the beat note signal S 1 . The difference between the beat signals S 1 and S 2 is only sensitive to timing variations and provides the clock signal AS 2 used for sampling the interferogram. Full size image Each filtered beat note signal can be considered as a time-stretched sampled waveform of an optical comb line. Any relative timing variation δ t shifts the interferometric signal by the stretched amount s δ t . If such a time-shifted beat note is used as a clock signal to trigger the data acquisition, it would correct for timing fluctuations automatically if the pulses were only subject to timing variations. However, frequency combs also produce unintended variations δφ of the phase difference between pump and probe pulse. These phase variations δφ are directly imprinted onto each frequency component of the detected signal. To correct for such phase fluctuations, the signal of the sampling detector is multiplied electronically with the beat note signal at f a . The difference in frequency between the beat signals at f a and f b is immune to common phase variations δφ and can provide the required adaptive clock signal, which compensates for timing variations. Experimental set-up In an experimental implementation of the scheme (see Fig. 2 for a detailed sketch), two free-running commercial femtosecond erbium-doped fibre lasers emitting in the 1,550-nm region are used. Their repetition frequencies are 100 MHz and differ by about 350 Hz. The experimental set-up is placed in a basic laboratory environment without air-conditioning system, vibration isolation or dust protection. Each free-running femtosecond erbium-doped fibre laser has two fibred output ports. 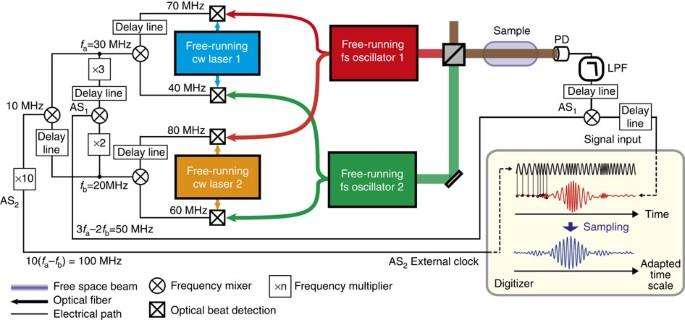Figure 2: General sketch of adaptive dual-comb spectroscopy. The output of a free-running femtosecond (fs) erbium-doped fibre laser is combined with that of a second free-running fs Er-doped fibre laser with a slightly different repetition frequency. Both beams probe the sample. Their temporal interference pattern is recorded with a fast photodetector (PD), filtered (LPF), mixed with the first adaptive signal and digitized. Each fs laser simultaneously beats with two independent narrow linewidth continuous-wave free-running erbium fibre lasers to isolate single longitudinal modes of each fs laser. Each pair of beating signals with a given cw laser is electronically mixed to produce an electric signal reporting the relative fluctuations between two modes of the two combs, at a frequencyfaandfb, respectively. These signals are frequency multiplied and mixed according to a manner described in the Methods section. They produce two adaptive signals AS1and AS2. The first adaptive signal AS1is mixed with the interferometric signal to compensate mainly for the phase variations while the second adaptive signal AS2serves as the external clock signal for data acquisition and accounts for the timing variations only. Figure 2: General sketch of adaptive dual-comb spectroscopy. The output of a free-running femtosecond (fs) erbium-doped fibre laser is combined with that of a second free-running fs Er-doped fibre laser with a slightly different repetition frequency. Both beams probe the sample. Their temporal interference pattern is recorded with a fast photodetector (PD), filtered (LPF), mixed with the first adaptive signal and digitized. Each fs laser simultaneously beats with two independent narrow linewidth continuous-wave free-running erbium fibre lasers to isolate single longitudinal modes of each fs laser. Each pair of beating signals with a given cw laser is electronically mixed to produce an electric signal reporting the relative fluctuations between two modes of the two combs, at a frequency f a and f b , respectively. These signals are frequency multiplied and mixed according to a manner described in the Methods section. They produce two adaptive signals AS 1 and AS 2 . The first adaptive signal AS 1 is mixed with the interferometric signal to compensate mainly for the phase variations while the second adaptive signal AS 2 serves as the external clock signal for data acquisition and accounts for the timing variations only. Full size image The ports that emit an average power of about 20 mW are used for the dual-comb spectroscopy when the other ports (about 10 mW) are generating the two adaptive signals AS 1 and AS 2 . For adaptive signal generation, each femtosecond laser independently beats with two free-running continuous-wave erbium-doped fibre lasers that emit at 1,534 and 1,557 nm, respectively. Two beat notes f cw − f 1, n and f cw − f 2, n are produced, thus isolating one line of each of the two femtosecond lasers. The electric signals ( Fig. 3 ) are filtered and delay lines adjust the timing between the beat signals. The two beat notes are electronically mixed so that the contribution of the continuous-wave laser cancels to generate the signal f a = f 1, n − f 2, n . We produce two such beat notes between individual comb lines from the two combs, with frequencies f a = f 1, n − f 2, n and f b = f 1,m − f 2,m . In our experiments, their values are 30 and 20 MHz, respectively. 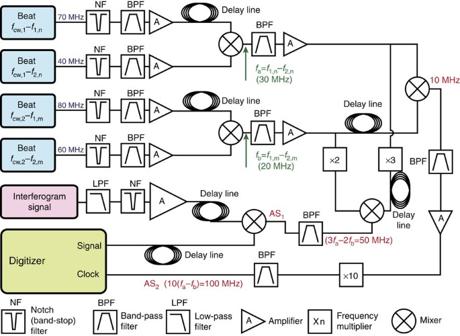Figure 3: Generation of the adaptive signals. This figure details the processing of the electronic analogue signals after the detection of the optical beats. The adaptive signals AS1and AS2are generated from the proper combination of four beat notes between comb lines and continuous-wave lasers. See text for further information. The filters were purchased from Minicircuits, K&L Microwave and KR Electronics; the amplifiers from Minicircuits and Miteq, the frequency multipliers from Wenzel Associates Inc. and the mixers were from Minicircuits. Figure 3: Generation of the adaptive signals. This figure details the processing of the electronic analogue signals after the detection of the optical beats. The adaptive signals AS 1 and AS 2 are generated from the proper combination of four beat notes between comb lines and continuous-wave lasers. See text for further information. The filters were purchased from Minicircuits, K&L Microwave and KR Electronics; the amplifiers from Minicircuits and Miteq, the frequency multipliers from Wenzel Associates Inc. and the mixers were from Minicircuits. Full size image As the radiofrequency spectrum spans the free spectral range 0– f /2, that is, 0–50 MHz, the signals at frequencies f a and f a − f b are not high enough to avoid aliasing. The first adaptive signal AS 1 is generated from a signal at frequency 3 f a −2 f b produced by a combination of frequency multipliers and mixers. The subsequent 50 MHz signal AS 1 is mixed with the interferometric signal before digitizing by the data acquisition board. The second adaptive signal AS 2 results from the frequency multiplication by a factor 10 of the beat signal at frequency f a − f b . A 100-MHz signal thus provides the adaptive clock signal AS 2 that is connected to the external clock input of the digitizing data acquisition board. We note that combs where the carrier–envelope offset cancels, as can be produced by difference frequency generation [28] , [37] would only require one adaptive signal [18] . The two 20 mW beams are combined to interrogate the sample and beat on a fast InGaAs photodiode. The time-domain interferometric signal exhibits a periodic succession of huge bursts every 1/Δ f when femtosecond pulses from the two lasers coincide. A low-pass filter essentially suppresses the non-interferometric signal at the pulse repetition frequency of 100 MHz. To synchronize the interferometric signal with the adaptive signals, one has to compensate for the delays induced by the different optical paths and the various electronic components. An electronic delay line is therefore inserted in the interferometric signal path. The interferometric electric signal is mixed with the first adaptive signal AS 1 . A low-noise 100-MHz-bandwidth amplifier with variable gain scales the filtered mixed signal to the full range of a 14-bit analogue-to-digital converter. This high-resolution digitizer, onboard a personal computer, has 65-MHz-bandwidth and sampling rate capabilities of up to 125 M samples s −1 . It is externally synchronized with the second adaptive clock signal AS 2 . The Methods section describes with additional details the experimental set-up. Stability of the free-running femtosecond lasers We have investigated the frequency stability of our free-running femtosecond lasers to characterize the instabilities we need to compensate for. The repetition frequency of each laser is measured with a frequency counter referenced to the 10-MHz signal of a hydrogen maser. The drift is nearly linear and amounts for about 7 mHz per second. Such drifts are mostly due to thermal fluctuations and are easy to suppress with a low-bandwidth feedback loop. The instability of an optical comb line is measured by an optical beat measurement with a continuous-wave erbium-doped fibre laser. The continuous-wave erbium-doped fibre laser is emitting at 1,542.5 nm and is stabilized against an ultra-low-expansion Fabry–Perot high finesse resonator. It has a linewidth of 1.5 Hz in a 1-Hz bandwidth and thermal drifts of its central position of 20 mHz s −1 (Predehl et al . [38] ). 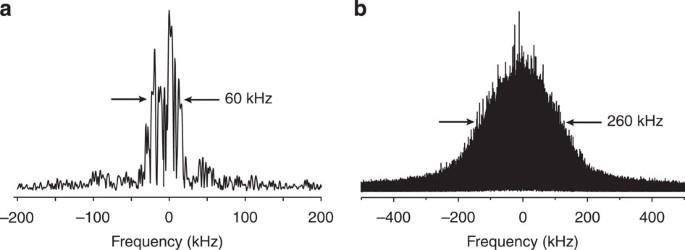Figure 4: Beat note of one comb line and a stabilized Hz-linewidth continuous-wave laser. (a) Over 467 μs, the time required for the acquisition of an interferogram, the width of the comb line is of the order of 60 kHz. This is much broader than the radiofrequency comb line spacing (344.9 Hz). (b) Over 1.3 s, the width of the comb line increases to 260 kHz. The spectra are displayed on a linear intensity scale. Figure 4 shows the beat notes at 460-μs ( Fig. 4a ) and 1.3-s ( Fig. 4b ) measurement times. Their linewidths are about 60 and 260 kHz, respectively. For longer times, the beat measurement drifts linearly by 6 kHz s −1 . As the linewidth and drift of the cw laser are negligible compared with these values, we can infer that we directly measure the width and instability of one optical comb line. The measured short-term comb linewidths are significantly too broad to achieve Doppler-limited dual-comb measurements in which the beat notes between pairs of comb lines should be narrower than a few hundreds of Hertz. Figure 4: Beat note of one comb line and a stabilized Hz-linewidth continuous-wave laser. ( a ) Over 467 μs, the time required for the acquisition of an interferogram, the width of the comb line is of the order of 60 kHz. This is much broader than the radiofrequency comb line spacing (344.9 Hz). ( b ) Over 1.3 s, the width of the comb line increases to 260 kHz. The spectra are displayed on a linear intensity scale. Full size image Experimental results The transmission spectrum by a 70-cm single-pass gas cell filled with 213 Pa of acetylene in natural abundance is recorded in the region of the ν 1 +ν 3 combination band. 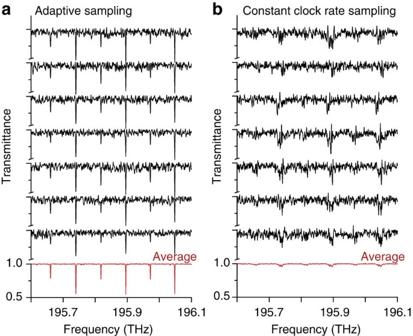Figure 5: Portions of experimental spectra of acetylene. (a) Zoom of a span of 0.5 THz of seven consecutive adaptive individual spectra (in black) and the average of 200 spectra (in red). Each individual spectrum is measured over a 14.5-THz span within 467 μs. (b) Spectra digitized at the constant clock rate of the data acquisition board and identical conditions than inaotherwise. The acetylene line profiles are strongly distorted and the drifts in the frequency scale do not allow for averaging. Figure 5 displays a 0.5-THz zoomed part of a 14.5-THz spectral span. Seven consecutive spectra are displayed. Each is measured within 467 μs with 1.1 GHz apodized resolution at a refresh rate of 350 Hz. The signal-to-noise ratio, estimated from the root-mean-square noise, in an individual spectrum is about 20. The individual spectra do not exhibit any phase error. The reproducibility of consecutive adaptive spectra permits efficient averaging, whereas free-running lasers without the adaptive sampling scheme produce strongly distorted spectra and do not allow for quantitative measurements or signal averaging. We compare ( Figs 6 and 7 ) a spectrum resulting of 200 averaging with a spectrum computed from the HITRAN database [39] as an illustration of the excellent quality of our experimental adaptive spectra. The good signal-to-noise ratio in the averaged adaptive spectrum clearly reveals the rotational lines of the ν 1 +ν 3 cold band, the ν 1 +ν 3 +ν 4 1 −ν 4 1 and ν 1 +ν 3+ ν 5 1 −ν 5 1 hot bands of 12 C 2 H 2 and even of the ν 1 +ν 3 cold band of 12 C 13 CH 2 , although its relative concentration is about a hundred times smaller. The level of the residuals between the adaptive spectrum and the calculated one is below 1.5%. Calibration against two molecular lines present in the adaptive spectrum sets the frequency accuracy on the other line positions to 10 MHz (relative accuracy: 5 × 10 −8 ) at 1 ms measurement time. The very good agreement between experimental and computed profiles shows the suitability of our technique for the measurement of line intensities or concentrations. Figure 5: Portions of experimental spectra of acetylene. ( a ) Zoom of a span of 0.5 THz of seven consecutive adaptive individual spectra (in black) and the average of 200 spectra (in red). Each individual spectrum is measured over a 14.5-THz span within 467 μs. ( b ) Spectra digitized at the constant clock rate of the data acquisition board and identical conditions than in a otherwise. The acetylene line profiles are strongly distorted and the drifts in the frequency scale do not allow for averaging. 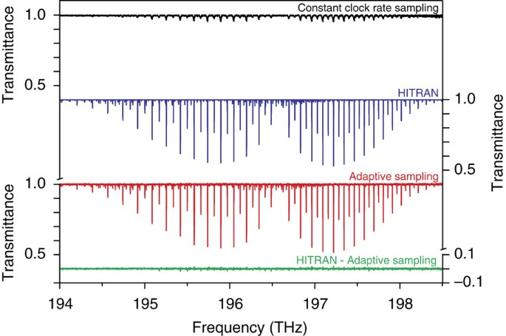Figure 6: Illustration of the quality of the adaptive sampling spectra. Experimental absorption spectra of12C2H2and12C13CH2sampled at adaptive and constant clock rates, respectively, are compared with a spectrum computed from the line parameters available in the HITRAN database39. The 70-cm-long cell is filled with 213 Pa of acetylene. Both experimental spectra are measured with free-running fs lasers in identical conditions except for the data acquisition clock. The difference in repetition frequencies between the two free-running fs lasers is set to 344.9 Hz. Two hundred consecutive spectra with an apodized resolution of 1.1 GHz, each measured within 467 μs, are averaged, resulting in a total measurement time of 93 ms and a total experimental time of 580 ms. The agreement of the experimental adaptive spectrum with the computed spectrum from the12C2H2and H12C13CH line parameters of the HITRAN database confirms the suitability of our technique for measurements with Doppler-limited resolution. When sampled at the constant clock rate of the digitizing data acquisition board, the spectrum is strongly distorted owing to the relative fluctuations of the repetition frequency and carrier–envelope phase slips of the fs lasers. This lowers the sensitivity and scrambles the spectral features. Full size image Figure 6: Illustration of the quality of the adaptive sampling spectra. Experimental absorption spectra of 12 C 2 H 2 and 12 C 13 CH 2 sampled at adaptive and constant clock rates, respectively, are compared with a spectrum computed from the line parameters available in the HITRAN database [39] . The 70-cm-long cell is filled with 213 Pa of acetylene. Both experimental spectra are measured with free-running fs lasers in identical conditions except for the data acquisition clock. The difference in repetition frequencies between the two free-running fs lasers is set to 344.9 Hz. Two hundred consecutive spectra with an apodized resolution of 1.1 GHz, each measured within 467 μs, are averaged, resulting in a total measurement time of 93 ms and a total experimental time of 580 ms. The agreement of the experimental adaptive spectrum with the computed spectrum from the 12 C 2 H 2 and H 12 C 13 CH line parameters of the HITRAN database confirms the suitability of our technique for measurements with Doppler-limited resolution. When sampled at the constant clock rate of the digitizing data acquisition board, the spectrum is strongly distorted owing to the relative fluctuations of the repetition frequency and carrier–envelope phase slips of the fs lasers. This lowers the sensitivity and scrambles the spectral features. 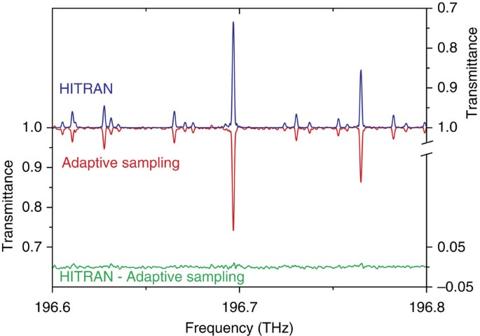Figure 7: Zoom of a 0.2-THz portion of the spectra. The adaptive experimental spectrum and the spectrum computed from the HITRAN data shown inFig. 6, together with the residuals, are expanded both in the x and y scales to better appreciate the high-resolution details. Full size image Figure 7: Zoom of a 0.2-THz portion of the spectra. The adaptive experimental spectrum and the spectrum computed from the HITRAN data shown in Fig. 6 , together with the residuals, are expanded both in the x and y scales to better appreciate the high-resolution details. Full size image Rather than averaging over several spectra, one can continuously record interferometric signals over a longer time period. In this way, it becomes possible to resolve the individual comb lines and thus to demonstrate that the coherence between the two femtosecond lasers is reconstructed during the measurement time. An interferogram is recorded in 2.7 s with 268 × 10 6 samples. The number of samples is limited by the memory of the data acquisition board. As the difference of repetition frequency of the lasers is set to 350 Hz, the interferogram comprises a continuous sequence of 945 bursts, each forming one of the individual interferograms used for Figs 6 and 7 . 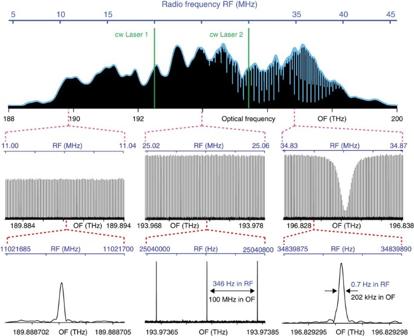Figure 8: Adaptive spectrum spanning 12 THz with resolved comb lines. The spectrum across the entire domain of emission of the erbium-doped fs fibre lasers exhibits 120,000 well-resolved individual comb lines. The measurement time is 2.7 s. It reveals several acetylene profiles shaping the discrete comb line intensities. The frequency of the continuous-wave lasers used in the production of the adaptive signals is indicated in green in the upper row of the figure. In the two lowest rows, different degree of zooms in three different spectral regions well apart from these two frequencies isolate the individual comb lines and prove that the coherence between the two combs is maintained over the time of the measurement. Figure 8 shows the resulting spectrum of acetylene spanning over 12 THz. The 120,000 individual comb lines are resolved across the full spectral span and their apodized instrumental linewidth is 202 kHz in the optical domain (0.7 Hz in the radiofrequency domain), although the resolution in the spectrum is limited by the comb line spacing f (here 100 MHz). Such resolution is sufficient to sample most of infrared molecular profiles at room temperature in the gas, liquid or solid phases. In comparison, a Michelson-based Fourier transform spectrometer would record a similar spectral domain, with 10 5 spectral elements and a resolution at best of the order of 100 MHz, in several hours. Figure 8: Adaptive spectrum spanning 12 THz with resolved comb lines. The spectrum across the entire domain of emission of the erbium-doped fs fibre lasers exhibits 120,000 well-resolved individual comb lines. The measurement time is 2.7 s. It reveals several acetylene profiles shaping the discrete comb line intensities. The frequency of the continuous-wave lasers used in the production of the adaptive signals is indicated in green in the upper row of the figure. In the two lowest rows, different degree of zooms in three different spectral regions well apart from these two frequencies isolate the individual comb lines and prove that the coherence between the two combs is maintained over the time of the measurement. Full size image Our adaptive scheme sufficiently compensates for the short-term relative fluctuations of the femtosecond lasers at any optical frequency. In this demonstration, all lasers are free running but their relative coherence is reconstructed in real time. In comparison with the width of molecular Doppler-broadened lines, the drift of the lasers is however negligible. We thus demonstrate that high-quality molecular spectra down to Doppler-limited resolution may be recorded under such conditions. Importantly, these spectra are fully suitable for line profile and line intensities measurements within a reasonable accuracy of about 5%. Therefore, the instrument is suitable for optical diagnostics in a variety of applications. Using free-running lasers has, however, the drawback not to allow for self-calibration of the frequency scale. The calibration must be performed against literature-known molecular lines present in the spectra. If absolute direct frequency calibration via the frequency combs or high accuracy in the measurements of narrow, for example, sub-Doppler, line profiles is needed, the combs could be stabilized to a radiofrequency reference, as they often are in frequency metrology. This only avoids long-term drifts and enables self-calibration, but does not improve the quality of the individual spectra. The adaptive sampling scheme can still be applied to compensate for the laser short-term instabilities. Although radiofrequency locking of the combs alone is not a possible alternative for dual-comb spectroscopy, it would expand the range of applications of adaptive sampling to precision spectroscopy. For example, by tuning stepwise the carrier–envelope offset of the combs from one acquisition to the other and interleaving spectra, sub-Doppler resolution determined by the interleaving step (and ultimately by the linewidth of the individual comb lines) becomes within reach and such scheme is currently under exploration with nonlinear two-photon excitation [31] . The possibility of using commercial femtosecond lasers or frequency comb systems without any sophisticated optical or electronic stabilization scheme considerably eases the implementation of a dual-comb spectrometer and should prompt new applications to real-time spectroscopy and sensing. The adaptive scheme and the averaging could also take advantage of digital sampling processors onboard the data acquisition system. The resulting advantage would be to reduce the size of the data files stored on the computer hard drive. It similarly brings suitable real-time processing, as demonstrated [27] after release of a preprint of the present work. In conclusion, through our demonstration of an accessible and robust technique of dual-comb spectroscopy with free-running femtosecond lasers, the recording of distortion-free spectra with Doppler-limited resolution over the full emission bandwidth of a femtosecond oscillator within a few hundreds of microseconds becomes feasible to scientists and engineers unfamiliar with the sophisticated tools of ultra-stable lasers. The key feature of dual-comb spectroscopy, the very short measurement time, is kept optimal. Detailed experimental set-up Figure 2 displays the technical scheme for the realization of the principle sketched in Fig. 1 . Two similar commercial mode-locked Er-doped fibre lasers (C-Fiber, MenloSystems GmbH) have their emission centred at 193 THz (1,550 nm) with a span of about 12 THz. The repetition frequency of the pulses is about 100 MHz. The repetition frequencies can be adjusted by moving a cavity mirror mounted on a motorized translation stage and a piezoelectric transducer. The difference of the repetition frequencies of the two lasers is chosen to be 350 Hz, a value imposed by the Nyquist criterion to avoid aliasing. Each laser has two fibred output ports. The first one with an average output power of 20 mW is used for the spectroscopy experiment, whereas the second one with an average output power of 10 mW is used to generate the adaptive signals AS1 and AS2. For the generation of the adaptive signals, we need to produce two beat signals between pairs of comb lines, one from each comb. We first isolate independently four individual comb lines, two from each comb. Free-running continuous-wave erbium-doped fibre lasers (Koheras Adjustik E15, NKT Photonics, with a claimed free-running linewidth of 1 kHz at 125 μs) emitting at 1,534 and 1,557 nm, respectively, serve as local oscillators. The narrow line spacing of the femtosecond lasers, of 100 MHz, does not indeed permit the use of an optical filter. The procedure to measure the beating signal between one of the femtosecond lasers and one of the continuous-wave lasers is the following: the beam of the femtosecond laser is superimposed to that of the continuous-wave laser with free space optical components. A short grating disperses coarsely the beam to avoid excess radiation outside the frequency range of the continuous-wave laser to impinge the detector. The beam spectrally centred on the frequency of the continuous-wave laser is focused onto a fast amplified InGaAs photodiode (FPD310-F, Menlosystems GmbH). Adjusting the polarization of each beam with a combination of half-wave plates and polarizing beam splitter makes it possible to optimize the signal-to-noise ratio of the beat note. The processing of the electronic signals after detection of the optical beats is detailed in Fig. 3 . A Notch filter rejects the strong 100-MHz signal of the repetition frequency of the femtosecond laser. The beat note is further band-pass filtered and amplified. Each cw laser individually beats with each comb and in total, we produce four such beat notes with a frequency ( f cw,1 − f 1, n , f cw,1 − f 2, n , f cw,2 − f 1, m , f cw,2 − f 2, m , respectively) smaller than 100 MHz and a signal-to-noise ratio higher than 30 dB. Two beat notes of frequency f cw,1 − f 1, n and f cw,1 − f 2, n , respectively, involving the same cw laser are electronically combined. The contribution of the continuous-wave laser cancels to generate the beat note between individual comb lines of frequency f a = f 1, n − f 2, n . Before electronically mixing the two signals, we need to adjust their timing as the different electronic components induce phase shifts. This is currently achieved by introducing passive delay lines (DB64, Stanford Research Systems). The delay induced by each individual component has been experimentally measured before assembling the set-up. The signal of frequency f a is again filtered and amplified. We produce two such beat notes between individual comb lines from the two combs, with frequencies f a = f 1, n − f 2, n and f b = f 1,m − f 2,m . In this experiment, their values are 30 and 20 MHz, respectively. As already explained in the main text of the article, the radiofrequency spectrum spans the free spectral range 0− f /2, that is, 0–50 MHz, the signals at frequencies f a and f a − f b are not high enough to avoid aliasing. The first adaptive signal AS 1 is generated from a signal at frequency 3 f a −2 f b produced by a combination of frequency multipliers, band-pass filters and mixers. The subsequent 50 MHz signal AS 1 is mixed with the interferometric signal before digitizing by the data acquisition board. The second adaptive signal AS 2 results from the frequency multiplication by a factor 10 of the beat signal at frequency f a − f b . A 100-MHz signal thus provides the adaptive clock signal AS 2 that is connected to the external clock input of the digitizing data acquisition board. For the spectroscopic interrogation, the two 20-mW output ports of the femtosecond lasers are combined on a 50–50 beam splitter. The combined beam passes through a home-made single pass 70-cm-long cell filled with 213 Pa of acetylene in natural abundance and is focused onto an InGaAs photodiode (1623, Newfocus). Low-pass filtering limits the bandwidth of the interferometric signal to the useful free spectral range (0–50 MHz) and suppresses the non-interferometric signal at the pulse repetition frequency of 100 MHz. To synchronize the interferometric signal with the adaptive signals, one has to compensate for the delays induced by the different optical paths and the various electronic components. An electronic delay line (Allen Avionics Inc.) is therefore inserted in the interferometric signal path. This delay line would require to be replaced in the future as it was found to induce low-pass filtering and attenuation. The interferometric electric signal is mixed with the first adaptive signal AS 1 . A low-noise 100-MHz-bandwidth amplifier with variable gain (DHPVA-100, Femto GmbH) scales the filtered mixed signal to the full range of an analogue-to-digital converter. The digitizer (ATS9440, AlazarTech) has 65-MHz-bandwidth and sampling rate capabilities of up to 125 M samples per s. Its specified dynamic range is 14 bits; however, the effective number of bits is limited by the converter noise to 9.54. We estimate the temporal jitter induced by the digitalization to 2 ps, which may be a reason for residual phase errors in the spectra. The digitizer possesses an external clock input, which makes it possible to synchronize the data acquisition with the second adaptive clock signal AS 2 . The internal memory of the digitizer is 2 28 (268 × 10 6 ) samples, which currently limits the duration of an acquisition at a sampling rate of 100 MHz to 2.7 s. Once the acquisition sequence is completed, the interferogram is stored on the computer hard drive. A set of computer programs Fourier-transforms the interferograms and help in the treatment and analysis of the resulting spectra. Fast Fourier transform of large data sets is performed with a choice of apodization functions. For representation, the spectrum is interpolated by zero-filling of the interferogram. Currently, the time needed for Fourier transforming, with a personal computer, an interferogram of 2 30 samples (2 28 of interferogram data, completed with zero-filling) is 120 s. We do not identify the current maximum number of samples as a limitation. Data acquisition boards with a larger memory are readily available. However, within the present 2.7 s acquisition time, we already achieve an instrumental width of the comb lines of 202 kHz, 500-fold better than the actual resolution in the spectrum, which is determined by the 100-MHz line spacing of the comb. Our demonstration primarily shows the robustness of our technique of adaptive sampling in reconstructing the coherence between the two combs and is aimed at Doppler-limited spectroscopy. We also anticipate that to fully benefit from longer acquisition times, the laser combs would need to be stabilized to a radiofrequency clock. On time scales of a few tens of seconds, the fluctuation of the combs is such that the frequency of the adaptive signals drifts out of the bandwidth of the filtering electronics. With stabilized combs, reaching an actual resolution of the order of 200 kHz in dual-comb spectroscopy would require to measure a sequence of 500 interferograms with different comb line positions, amounting in total of 3 × 10 11 samples, and to reconstruct a posteriori the high-resolution spectrum by interleaving the individual spectra with resolved comb lines. While the perspective of sub-Doppler dual-comb broad spectral bandwidth spectroscopy is certainly exhilarating, it will also require extensive efforts in data treatment and analysis techniques, and achieving a 200-kHz resolution over a 10-THz span would already represent a major achievement. How to cite this article: Ideguchi, T. et al . Adaptive real-time dual-comb spectroscopy. Nat. Commun. 5:3375 doi: 10.1038/ncomms4375 (2014).